The WEIZMASS spectral library for high-confidence metabolite identification Annotation of metabolites is an essential, yet problematic, aspect of mass spectrometry (MS)-based metabolomics assays. The current repertoire of definitive annotations of metabolite spectra in public MS databases is limited and suffers from lack of chemical and taxonomic diversity. Furthermore, the heterogeneity of the data prevents the development of universally applicable metabolite annotation tools. Here we present a combined experimental and computational platform to advance this key issue in metabolomics. WEIZMASS is a unique reference metabolite spectral library developed from high-resolution MS data acquired from a structurally diverse set of 3,540 plant metabolites. We also present MatchWeiz, a multi-module strategy using a probabilistic approach to match library and experimental data. This strategy allows efficient and high-confidence identification of dozens of metabolites in model and exotic plants, including metabolites not previously reported in plants or found in few plant species to date. Metabolite annotation in untargeted, metabolomics analysis is a critical but yet unsolved problem in mass spectrometry (MS)-based metabolomics [1] , [2] . It is particularly important in studies of complex metabolic matrices such as those produced by plants. While over 200,000 chemical structures have been attributed to plants to date, this number likely represents only a small part of the global plant metabolic repertoire [3] , and it is estimated that a single plant could be producing up to 15,000 metabolites [4] . The majority of these metabolites represent specialized metabolites (or secondary metabolites) that accumulate to high levels in certain plant families or species. These metabolites possess a myriad of biological activities and serve as a base for traditional and modern drugs, as well as a source of nutraceuticals and cosmetics. The currently most wide-spread technology for metabolomics assays is high-resolution MS that is typically coupled with liquid chromatography (LC–MS) [5] , [6] , [7] . The availability of authentic standards, or carrying out metabolite purification followed by nuclear magnetic resonance (NMR) analysis, are crucial for high-confidence level metabolite identification as it is largely impossible to infer unambiguous structure of metabolites using only LC–MS. This holds true even with MS instruments providing the highest mass accuracy [8] . As a result, metabolomics assays suffer from relatively low discovery rate and even false identifications, and only a few percent of the detected metabolites can be assigned a confident, unambiguous identity [9] . The naive, straightforward, approach for feature annotation in LC–MS analysis is by matching each unique mass signal to the mass of all theoretically possible and relevant metabolites. Such a method is inefficient, primarily due to the high number of potential mass isomers and the considerable amount of instrumental noise, which both contribute to high rates of false identifications and to low discovery rates [10] , [11] . Another major reason for poor overall discovery rates is the low coverage of public or commercial LC–MS spectra libraries that are based on accurately curated and confidently identified plant metabolites. LC–MS spectral libraries representing unequivocally assigned, purified or synthesized plant metabolites reported to date [12] , contain a relatively limited set of records which are based on injections of authentic chemical standards (for example, the ReSpect database (DB) [13] ). Consequently, a boost to the number of structures currently available in MS databases is highly desired. High-confidence, metabolite identification (so called metabolomics standards initiative (MSI) level 1 (ref. 2 )) requires comparison of two or more orthogonal properties of a chemical standard to the same properties observed for the metabolite of interest, analysed under identical analytical conditions [2] . However, even at this level of confidence, some cases of ambivalence are possible; notably, stereoisomers are not always distinguishable even with the finest chromatographic separation methods and structural determination by NMR spectroscopy must therefore be used. For that reason, new criteria for reporting confidence in metabolite identification have recently been proposed, evolving a more elaborated mechanism for describing annotated metabolites [14] , [15] . Generating a comprehensive mass spectra library from highly pure metabolite standards, isolated from an extensive repertoire of plant species, is one possible strategy to advance metabolite annotation in plant metabolomics. Once such a library is generated it should be coupled to computational tools that allow efficient and accurate matching of experimental to library LC–MS data. The current methodologies for such matching include the use of MS fragmentation trees, MS 2 mass spectral tags coupled with matching databases and computational fragmentation spectra [16] , [17] , [18] , [19] , isotope patterns for molecular formula decomposition [20] , and chromatographic retention time (RT) prediction models [21] , [22] , together with streamlining tools such as MZmine, Metabo-Analyst and XCMS online [23] , [24] , [25] . Here a comprehensive set of more than 3,500 different highly pure, structurally verified, plant metabolites (mostly specialized metabolites) was used for generating a structurally diverse LC–MS spectra library, termed WEIZMASS. A complementary computational method that automatically constructs such a spectral library has been developed, as well as a dedicated multi-module computational approach, termed MatchWeiz, that allows interrogating the WEIZMASS spectra against a given experimental LC–MS data. We demonstrate the application of this new strategy to confidently identify several dozens of metabolites from the extracts of three different plant species, including model as well as exotic plants. Furthermore, structures that were never published and associated with a particular living organism or those found in only single or several species to date are detected and identified in the studied plant extracts. The WEIZMASS library of highly pure chemical standards To generate a comprehensive reference mass spectra library of plant-derived metabolites we used a set of 3,540 highly pure standard metabolites. This repertoire of metabolites was isolated by AnalytiCon Discovery ( www.ac-discovery.com ) from more than 1,400 different plant species and includes known, as well as ∼ 40% metabolites that are not present in the comprehensive Dictionary of Natural Products ( www.dnp.chemnetbase.com ) and were extracted and characterized for the first time in any living organism. Chemometric analysis of the library based on molecular fingerprints and the Tanimoto similarity index [26] reveals high structural diversity within the library compounds ( Fig. 1a ): 73.1% of the compounds share co-similarity indices lower than 0.4 and 97.6% share similarity values lower than 0.7. This reflects the large biological and taxonomic scope of the library, as well as the natural diversity of plant secondary metabolism. 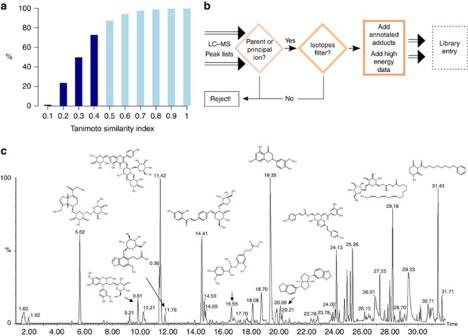Figure 1: Generating the WEIZMASS standard-based reference library. (a) The diversity of the reference library is summarized by a histogram showing the cumulative Tanimoto similarity index26between all library metabolites. Each bar represents the percent of library metabolites pairs having up to the specified Tanimoto similarity index value. As about 50% of the library metabolites have similarity indices lower than 0.3 and over 80% are in the lower than 0.5 range, the library can be considered very structurally diverse. (b) An outline of the software which automatically creates the reference library (see Methods section andSupplementary Figs 2 and 3). (c) Example chromatogram of a pool of chemical standards analysed by high-resolution MS in the NI mode. The chemical structures of 11 library metabolites are given above the corresponding peaks. Figure 1: Generating the WEIZMASS standard-based reference library. ( a ) The diversity of the reference library is summarized by a histogram showing the cumulative Tanimoto similarity index [26] between all library metabolites. Each bar represents the percent of library metabolites pairs having up to the specified Tanimoto similarity index value. As about 50% of the library metabolites have similarity indices lower than 0.3 and over 80% are in the lower than 0.5 range, the library can be considered very structurally diverse. ( b ) An outline of the software which automatically creates the reference library (see Methods section and Supplementary Figs 2 and 3 ). ( c ) Example chromatogram of a pool of chemical standards analysed by high-resolution MS in the NI mode. The chemical structures of 11 library metabolites are given above the corresponding peaks. Full size image Comparison with other high-resolution plant MS libraries We compared WEIZMASS with the high-resolution MS spectra data of phytochemicals in the ReSpect DB [13] . In terms of size, the WEIZMASS library has 3,308 unique chemical structures related to 1,785 chemical formulas, while 465 chemical structures and 397 chemical formulas could be found in the ReSpect DB ( Supplementary Table 1 ). In addition, a very low number of metabolites (roughly 3%) of the WEIZMASS library have identical chemical structures in the ReSpect DB, emphasizing the novelty of the presented data. We further compared the WEIZMASS library with the GNPS (Global Natural Products Social Molecular Networking) database, which is not exclusive to either plant or natural products. The ‘PRESTWICK PHYTOCHEM’ GNPS plant product library currently contains 140 unique chemical structures, and additional three non-plant specific natural products libraries (the ‘NIH-NATURALPRODUCTSLIBRARY’, the ‘FAULKNERLEGACY’ and the ‘GNPS LIBRARY’) currently contain 1,941 unique SMILES strings (corresponding with unique chemical structures, of which only 1,242 were readable and could be processed; see Methods section). These libraries cannot, however, be directly compared with the WEIZMASS library, as we could not determine how many of their entries are plant related and have an MS spectra derived from a chemical standard. Regardless, we found no overlap between any of the GNPS libraries and the WEIZMASS library, and the highest Tanimoto similarity index between any WEIZMASS metabolite and the mentioned GNPS libraries was 0.17, implying very distinct chemical spaces. Finally, we compared the WEIZMASS library with the Spektraris repository [27] , which is dedicated to identification of compounds produced in plants. The Spektraris DB contains 487 unique chemical structures and 422 unique chemical formulas, compared with 3,308 unique chemical structures and 1,785 unique chemical formulas in the WEIZMASS library. Again, we found no overlap between the Spektraris DB and the WEIZMASS library, and the highest Tanimoto similarity index between the libraries was 0.18, indicating very distinct chemical spaces. Pipeline to construct MS libraries from chemical standards The mass spectra of individual molecules in the collection were acquired using a high-resolution quadrupole time-of-flight (QTOF)-MS instrument in the electrospray (+) and (−) ionization modes (that is, the positive (PI) and negative (NI) ionization modes; Fig. 1c ). To reduce the intensive analysis time of running individual standards, the spectral library (that is, WEIZMASS) was acquired over two batches consisting of 177 pools of 20 standards. Composition of the pools was determined based on the expected RT of each standard, to reduce the chances of co-eluting compounds. Quality control samples and RT correction pools were included in each batch to correct for batch effects. A second, high-energy channel, which typically produces more mass fragments was also added using the ramping of MS collision energies (MS E mode with energy ramp [28] ). This provided additional peak fragment data to the library. We subsequently developed a computational method in which the LC–MS experimental data are automatically converted into a digital reference library using a software tool. This enables us to supersede the size and speed limit posed by manual labour of a human specialist, while maintaining reliability. An outline of the process for generating the WEIZMASS reference library and an example pool of chemical standards are presented ( Fig. 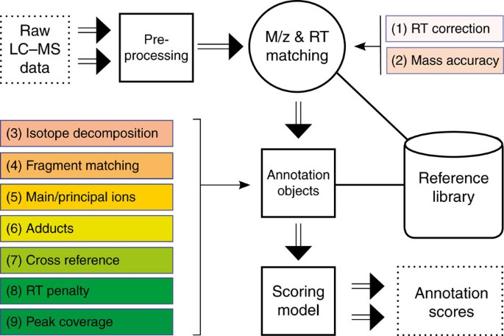Figure 2: The MatchWeiz software annotation workflow. Raw LC–MS data are preprocessed to produce peak tables. Next, the input data are concatenated through a preliminarym/zand RT matching function, getting inputs from modules (1) and (2), which relates peak groups from the input data to library entries. Modules (3)–(9) then process particular aspects of the data and return their results to an annotation object containing the obtained information regarding putative hits. Information is finally evaluated by the scoring model, which gives each annotation a score based on all available data. 1b,c , Supplementary Figs 2–4 and Supplementary Table 2 ). The automatic processing of the pools resulted in reference spectra of 2,741 and 2,724 unique metabolite in the PI and NI modes, respectively. 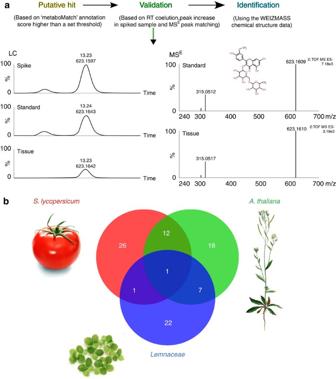Figure 3: Validation and high-confidence identification of metabolites. (a) Putative hits are experimentally confirmed using three consecutive injections consisting of the endogenous tissue samples, the tissue samples spiked with the corresponding chemical standards and the pure chemical standards. (b) A Venn diagram presenting the total counts of annotated metabolites for tomato (red),A. thaliana(green) and members of the Lemnaceae family (blue). Tomato image courtesy of Fir0002/Flagstaffotos under GFDL v1.2 license.Arabidopsisimage courtesy ofhttp://delta-intkey.com/angio/www/crucifer.htm(ref.49). The photo of Lemna plant was produced in-house. In total, 3,309 unique metabolite entries (out of 3,540 standards injected to LC–MS) were detected in the two ionization modes ( Supplementary Table 3 ). The loss of 231 chemical standards was mostly a result of weak ionization and lower than expected amount of the chemical standard. Masking effect of noise peaks in the pools of the chemical standards (for example, Fig. 1c ) and software retrieval issues during the preprocessing and library creation steps might also explain part of the loss in compound detection. In addition, 18 metabolites (about 0.5% of the library) have a molecular weight higher than 1,500 Da, which exceeded the mass range settings of our measurements. To test the quality of the automatically generated library we randomly chose several library pools of 20 metabolites each and evaluated manually the performance of the automatically inserted library entries for each metabolite. The evaluation indicates that the software-created library is on par with manual curation: considering the true insertions of metabolites into the library, the software achieved a mean sensitivity (or true positive rate) of 0.97 for the NI mode and 0.94 for the PI mode. 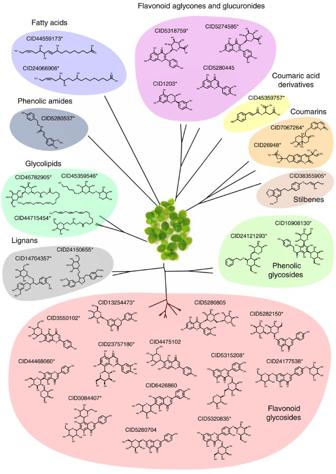Figure 4: Clustering by structural similarity of identified metabolites detected in members of the Lemnaceae family. The Tanimoto similarity index26was used to calculate the similarity between the identified metabolites based on their molecular fingerprints (1,024 bits, binary). Metabolites marked with asterisks are either ‘never published in that plant species’, or ‘never published or associated with any organism’ (Supplementary Data 1–4). PubChem CIDs corresponding with each metabolite are given next to the chemical structure. See also ‘Clustering of identified metabolites by structural similarity’ in the Methods section. Considering the true rejections of missing metabolites from the library, the software achieved a mean specificity (or true negative rate) of 0.95 for the NI mode and 0.87 for the PI mode (full evaluation results are presented in Supplementary Table 4 ). The purity of chemical standards is crucial for the successful application of the automatic method. For example, in a very particular case, the chemical standard of the flavonoid naringenin chalcone contained also its mass isomer naringenin. Since both metabolites typically elute at an almost identical RT and have an identical mass spectra, the automatic processing method erroneously switched between the two metabolites ( Supplementary Fig. 5 ). The MatchWeiz modular approach for metabolite annotation Matching experimental MS spectral data derived from complex matrices (for example, plant extracts) to a large spectral library of reference metabolites like WEIZMASS while minimizing false positive rates, requires a computational tool that will take an advantage of the various data features obtained from chromatography and high-resolution MS. To address this challenge, we developed a software (termed MatchWeiz), representing a multi-modular approach in which each feature of the data is independently processed and evaluated by a different computational module ( Fig. 2 ). MatchWeiz comprises nine modules, some of which were specifically developed while others represent new implementations of earlier work from our lab and others. These modules include the following: (1) RT correction—chromatographic shift correction using RT tags. This module corrects for systematic shifts in chromatography to improve matching observed RT to the values registered in the reference library; (2) mass error—an adaptive mass-to-mass matching using a mass error prediction model. This module optimizes mass-to-mass matching using statistics of the specific analytical instrument [29] ; (3) optimized isotope decomposition—using filters to reduce the size of the candidate list resulting from isotope decomposition methods [20] and using the filtered lists to evaluate chemical formula equivalence; (4) fragment matching—this module applies a rank-based model [30] for the matching of experimental mass fragments to fragments registered in the reference library; (5) main ions—evaluating the mass-to-mass matching of the molecular and/or the principal mass ions; (6) adducts—accounting for the presence of adduct ion species; (7) cross referencing MS ionization modes—scoring the correspondence between the two ionization modes based on complementary mass peaks; (8) RT penalty—RT penalty of matches with exceptional RT shifts; and (9) peak coverage—providing the fraction of peaks retrieved from the reference library ( Fig. 2 and Supplementary Note 1 for a complete description of the MatchWeiz software modules). Figure 2: The MatchWeiz software annotation workflow. Raw LC–MS data are preprocessed to produce peak tables. Next, the input data are concatenated through a preliminary m / z and RT matching function, getting inputs from modules (1) and (2), which relates peak groups from the input data to library entries. Modules (3)–(9) then process particular aspects of the data and return their results to an annotation object containing the obtained information regarding putative hits. Information is finally evaluated by the scoring model, which gives each annotation a score based on all available data. Full size image Evaluation of MatchWeiz retrieval rates To validate the results obtained by MatchWeiz we first evaluated its capacity to retrieve and identify a random set of 100 chemical standards from the WEIZMASS library that were spiked (separately, in each MS ionization mode) into a sample composed of Arabidopsis thaliana leaves and red stage tomato fruit skin extracts. We applied MatchWeiz to check how many of the spiked chemical standards could be retrieved successfully. The results were compared with the list of metabolites identified by human specialists who inspected manually each chromatogram in a targeted manner. The overall software retrieval rate was 174 out of 200 cases (100 chemical standards, injected in the PI and NI modes), compared with 183 out of 200 cases retrieved by human specialists. We assume that the 17 metabolites not detected manually had very low intensity peaks or were masked by the biological matrix. In the NI mode, the software retrieved 82 out of 89 metabolites detected by a human specialist (a 92.1 percent retrieval rate), and identified 6 (out of 11) metabolites not detected manually (that is, probably false annotations of other metabolites related to the biological matrix). In the PI mode, 92 out of 94 of the metabolites were retrieved (97.8%), and 3 out of 6 metabolites not found by manual identification were identified by the software. Overall, our computational approach resulted in high retrieval rates, very good overlap with manual detection results, but with a certain rate of false annotations, which also depended on the search parameters used. Training the MatchWeiz scoring model We next trained a scoring model that summarizes the output of the different modules to give a unified annotation score. The annotation score is based on the predicted probability for a true hit according to a logistic regression model (see Methods section). This approach enables us to weigh and summarize the different aspects of LC–MS data and to obtain a standardized software output. The interpretation of the scores can then be optimized for particular situations by the user (that is, maximize true discovery rate, or alternatively, minimize false matches). The initial scoring model was trained on the set of 100 spiked chemical standards described above, using the 174 cases of successfully retrieved metabolites as positive training examples. The annotation scores of the different computational modules were used as the predictive variables in the scoring model, and the predicted tags for each annotated metabolite were either ‘true’ (that is, one of the 174 cases of spiked chemical standards) or ‘unknown’ (that is, annotations originating from peaks related to the biological matrix). The scoring model was further retrained and optimized by validated library search results in extracts derived from three plant species: tomato ( Solanum lycopersicum ); A. thaliana ; and several species of the Lemnaceae family. Each putatively annotated metabolite with a score higher than a set threshold was experimentally validated, and the validated results were used to retrain the scoring function. Experimental validation for high-confidence identification (i.e.`MSI level 1' (ref. 2 )) was conducted by injecting the relevant pure chemical standard, spiking it into the extract sample and subsequently comparing both with the endogenous extract sample (expecting an increase in the spiked sample; Fig. 3a ). Figure 3: Validation and high-confidence identification of metabolites. ( a ) Putative hits are experimentally confirmed using three consecutive injections consisting of the endogenous tissue samples, the tissue samples spiked with the corresponding chemical standards and the pure chemical standards. ( b ) A Venn diagram presenting the total counts of annotated metabolites for tomato (red), A. thaliana (green) and members of the Lemnaceae family (blue). Tomato image courtesy of Fir0002/Flagstaffotos under GFDL v1.2 license. Arabidopsis image courtesy of http://delta-intkey.com/angio/www/crucifer.htm (ref. 49 ). The photo of Lemna plant was produced in-house. Full size image Metabolite identification in extracts of three plant species The currently available information regarding metabolite composition (particularly specialized metabolism) in the small, aquatic monocots of the Lemnaceae family is most limited. We used MatchWeiz to scan LC–MS data from samples of three members of the Lemnaceae family, namely Lemna gibba , Spirodela polyrhiza and Spirodela oligo ( Landoltia punctata ), which resulted in 31 identified metabolites of diverse chemical classes. Most of the identified metabolites are unique to the monocot Lemnaceae family, when compared with the investigated dicot, land plants ( Fig. 3b ). Only one identified metabolite was commonly shared among the three plant species (a lignan; PubChem ID 24150655, see Supplementary Data 1–3 for details on identified metabolites). Structural clustering of the identified metabolites ( Fig. 4 ) reveals a wide scope of chemical classes, as well as 26 (out of 31) metabolites, which to the best of our knowledge, are confidently identified in the Lemnaceae family for the first time ( Supplementary Data 1 ). Figure 4: Clustering by structural similarity of identified metabolites detected in members of the Lemnaceae family. The Tanimoto similarity index [26] was used to calculate the similarity between the identified metabolites based on their molecular fingerprints (1,024 bits, binary). Metabolites marked with asterisks are either ‘never published in that plant species’, or ‘never published or associated with any organism’ ( Supplementary Data 1–4 ). PubChem CIDs corresponding with each metabolite are given next to the chemical structure. See also ‘Clustering of identified metabolites by structural similarity’ in the Methods section. Full size image High-confidence metabolite identification (‘MSI level 1’ (ref. 2 )) is of great value in the fields of plant natural product chemistry and metabolomics. Yet, results providing such data (including specific chemical substitutions and positional isomers), are also critical for the discovery of novel pathways of specialized metabolism and the possibility of unravelling their corresponding genes and enzymes. For example, our analysis of Lemnaceae revealed high abundance of flavones (namely, apigenins and luteolins), which are typically present in monocots [31] . However, we also found flavonols in some of the species (for example, rutin, PubChem CID 5280805, that was detected only in L. punctata , indicating the likely presence of an active flavonol-3-hydroxylase enzyme in this particular strain [32] ). Further examination of the flavonoid profiles within the genus showed a clear differentiation between the two analysed Spirodela and L. gibba species; namely, only the Spirodela species contained both flavones and flavonols, whereas in the L. gibba species only flavones were identified. Two structural isomers identified in L. gibba : isoorientin (library compound NP-000286, PubChem CID6426860; see Supplementary Data 4 , pages 46–49); and 8-galactosyl-luteolin (library compound NP-001271, PubChem CID23757180; Supplementary Data 4 , pages 53–55) almost co-elute under the chromatographic conditions used. These isomers could be produced either through the activity of a single enzyme catalysing both glycosylation reactions or by two enzymes with different product specificity. From the enzymatic reaction perspective, only through high-confidence identification as performed here, the nature of the glycosyl substituent in the molecule and hence the glycosyl-donor substrate of the enzyme that catalyses the reaction, which in this case is an activated galactose, can be determined. Furthermore, some C- and O-diglycosides of flavonoids such as isovitexin-2″-O-arabinose (library compound NP-013098, PubChem CID44468060; Supplementary Data 4 , pages 87–90) were exclusively identified in the Spirodela species, indicating the presence of additional enzymes that catalyse reactions leading to more complex glycosylation patterns in the species. MatchWeiz was next used to scan the LC–MS data of 17 tomato ( S. lycopersicum ) extracts obtained from fruit (flesh and skin tissues from five stages of development), leaves (young, mature), buds, flower buds, open flowers, pollen and roots. Validation assays of the top hits obtained by MatchWeiz in both MS ionization modes resulted in highly confident MSI level 1 identification of 40 metabolites (including few stereo-isomers that could not be distinguished with the available analytical means). As in the case of the Lemnaceae family, clustering of the identified metabolites based on structural similarity ( Supplementary Fig. 14 ) shows the diversity of identified chemical classes, for example, flavonoids, fatty acids, lignans, organic acids, phenolic amides, phenolic glycosides, terpenoids and so on. Out of the 40 identified metabolites, only 19 have been previously reported in tomato, thus 21 metabolites (52.5%) have never been reported in this plant species and one of which has, to the best of our knowledge, never been published to exist in any organism (determined through search in public and in-house data, see ‘Determining the novelty of identified metabolites’ in the Methods section and Supplementary Data 5 ). We clustered experimental metabolic profiles according to abundance across five developmental stages in the flesh and skin tissues of tomato fruit. Metabolites belonging to the flavonoid glycosides and lignan chemical classes are relatively enriched in the fruit skin tissue, showing distinct abundance profiles across the five developmental stages. The profiles of the lignans (acanthoside B, and three unnamed lignans) show differential patterns of accumulation in the two fruit tissues ( Fig. 5 ). While flavonoid glycosides (particularly flavonols) accumulation in tomato fruit skin was described several times in the past [33] , [34] , this is the first report describing lignans in tomato. Both classes of metabolites are products of the phenylpropanoid pathway and our finding here suggests that, as is the case for the flavonoids, most of the lignan pathway is likely non-active in the fruit flesh tissue. 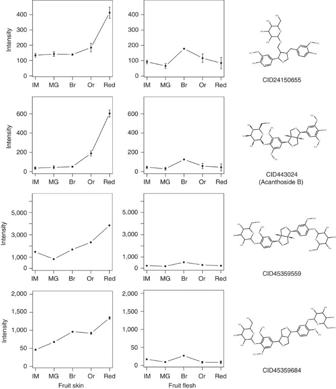Figure 5: Accumulation of lignans during tomato fruit development in skin and flesh tissues. Five developmental stages of tomato fruit: immature green (IG); mature green (MG); breaker (Br); orange (Or); and red (Red), are denoted on thexaxis, related to fruit skin (left plots) and fruit flesh (right plots). The mean values of LC–MS peak intensities are denoted on theyaxis, along with error bars denoting the s.e.m. (three biological replicates). The identified lignans show peaks of accumulation during the red fruit ripening stage in the fruit skin tissue, while levels of these lignans are relatively lower along all stages of fruit development in the fruit flesh tissue. Figure 5: Accumulation of lignans during tomato fruit development in skin and flesh tissues. Five developmental stages of tomato fruit: immature green (IG); mature green (MG); breaker (Br); orange (Or); and red (Red), are denoted on the x axis, related to fruit skin (left plots) and fruit flesh (right plots). The mean values of LC–MS peak intensities are denoted on the y axis, along with error bars denoting the s.e.m. (three biological replicates). The identified lignans show peaks of accumulation during the red fruit ripening stage in the fruit skin tissue, while levels of these lignans are relatively lower along all stages of fruit development in the fruit flesh tissue. Full size image The third plant species screened using MatchWeiz and the WEIZMASS library was the model plant Arabidopsis . We used the LC–MS data of 7 plant tissues (inflorescence, inflorescence leaves, young and mature leaves, closed buds, open flowers and silique) and confidently confirmed the identity of 38 metabolites. Twenty-one of the identified metabolites (55.2%) have, to the best of our knowledge, never been reported in this plant species and out of which four were, to the best of our knowledge, never published to exist in any organism ( Supplementary Data 6 ). The newly identified metabolites were clustered according to their abundance profiles together with a group of known specialized Arabidopsis metabolites. The results show co-expressed groups with correlated abundance profiles across different plant tissues ( Fig. 6 ). Structural clustering of the Arabidopsis metabolites based on similarity was also performed, as described for Lemnaceae and tomato above ( Supplementary Fig. 15 ). 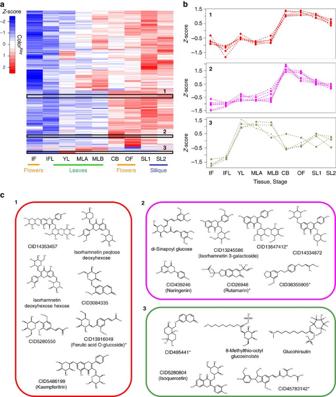Figure 6: Grouping of new and previously reported metabolites in the model speciesA. thaliana. (a) The heat map presents the relative intensity profiles of LC–MS peak groups. The samples (denoted in columns) were clustered according to tissues and developmental stages: inflorescence (IF); inflorescence leaves (IFL); young leaves (YL); mature leaves 3–4 and 7–8 weeks old (MLA and MLB respectively); closed buds (CB); open flowers (OF); and silique of 1 and 2 cm length (SL1 and SL2, respectively). Peak groups (denoted in rows) were clustered according to intensity profiles. Three metabolite clusters of interest are outlined in black. (b) The three metabolite clusters of interest are shown in detail. Metabolites are those reported for the first time inA. thalianaand ones previously assigned and reported in the species. (c) The chemical structures and PubChem CIDs corresponding with metabolite clusters inbare shown inside the colour boxes. See also ‘Clustering of chromatographic peaks by intensity profiles’ in the Methods section. Figure 6: Grouping of new and previously reported metabolites in the model species A. thaliana . ( a ) The heat map presents the relative intensity profiles of LC–MS peak groups. The samples (denoted in columns) were clustered according to tissues and developmental stages: inflorescence (IF); inflorescence leaves (IFL); young leaves (YL); mature leaves 3–4 and 7–8 weeks old (MLA and MLB respectively); closed buds (CB); open flowers (OF); and silique of 1 and 2 cm length (SL1 and SL2, respectively). Peak groups (denoted in rows) were clustered according to intensity profiles. Three metabolite clusters of interest are outlined in black. ( b ) The three metabolite clusters of interest are shown in detail. Metabolites are those reported for the first time in A. thaliana and ones previously assigned and reported in the species. ( c ) The chemical structures and PubChem CIDs corresponding with metabolite clusters in b are shown inside the colour boxes. See also ‘Clustering of chromatographic peaks by intensity profiles’ in the Methods section. Full size image Additional analysis of all identified metabolites in the three plant species according to botanical origin (see Supplementary Fig. 16 ) show a diverse distribution of identified metabolites over the phylogenetic tree representing the botanical origin of 671 (out of 790) plant genera represented in the WEIZMASS library. The phylogenetic analysis suggests that the possibility to identify new metabolites in any given plant species is not limited to the phylogenetic relatives of the investigated plant, but can originate from the full range of plant genera comprising the library. See `Analysis of identified metabolites by botanical origin' in the Methods section for further details. Comparison of MatchWeiz to other methods Unlike the proteomics field, where a solid reference in the form of true negative samples allows direct calculation of the false discovery rate [35] , the benchmarking of software in metabolomics studies is yet an unsolved issue. In metabolomics there are no clear standards to evaluate software annotation results, apart from experimental validations of each and every putative hit, which are only realistic if the list of putative software hits is relatively short. Therefore, the benchmark results presented here relate only to the list of MatchWeiz annotations, which were experimentally validated in a specific tissue (that is, tomato skin tissue). MatchWeiz was compared ( Supplementary Table 5 ) with the following: (i) an in-house software running a ‘naive’ search, where a minimal group of peaks with matching RT and m / z values to the library is considered an identified hit; and (ii) a commercial software, Progenesis QI ( http://www.nonlinear.com ), utilizing several orthogonal properties to evaluate a hit and using a scoring system which gives each property a partial score of 20 out of 100. All software were compared by the retrieval rates of the validated true hits, obtained using the same data, by the length of the overall candidate list for a particular software set-up and by the relative ranking position (RRP) [36] of the true candidate in individual cases. The evaluated candidate lists contain the results of the corresponding software after filtering by a score threshold (MatchWeiz, Progenesis QI) or ‘as-is’ (the ‘naive’ approach). Results of the comparison between MatchWeiz and the ‘naive’ approach show a clear dependence of the ‘naive’ approach on the search tolerance values and a large increase in the candidates list (from 180 to 840) when a good recall is obtained ( Supplementary Table 5 ). A large candidate list, such as produced by the ‘naive’ approach, represents a potentially high false discovery rate, and is generally impractical for experimental validation, thus eventually affecting the retrieval rate. On the other hand, the automatic estimation of search tolerance values with the multi-modular approach implemented in MatchWeiz, avoids issues of manually ‘guessing’ the optimal search tolerance parameters while providing a much smaller candidate list. We found that roughly 50% of MatchWeiz top-scoring results correspond with true hits, whereas in qualitative approaches such as the ‘naive’ search the situation is many times worse, since no priority can be given to the list of results. In addition, many top-scoring MatchWeiz candidates that do not confidently correspond with the chemical standard, and thus labelled as ‘false positives’, appear in many cases to be structural isomers of the true candidate. Such metabolites, having MS spectra closely related to that of the chemical standard, could potentially be regarded as lower-confidence (i.e. MSI level 2 or 3) hits. The comparison with Progenesis-QI was performed utilizing data obtained with a more accurate and sensitive high-resolution LC–MS instrument as compared with the instrument on which the core experiments in this study were performed. Thus, even though many more putative hits were detected, only previously validated results were taken into account. In comparison with Progenesis QI, MatchWeiz performed better both in terms of retrieval rates ( ∼ 50% higher) and in the length of the overall candidate list (approximately five times smaller). A reoccurring problem in annotation software results is that multiple annotations are often related to the same group of peaks. In this case, the more intricate scoring algorithm of MatchWeiz, which is based on a larger number of orthogonal properties than Progenesis QI, provided fewer multiple hits per peak group. The RRP, calculated for each of the retrieved metabolites ( Supplementary Table 5 ), demonstrates the advantage of MatchWeiz. While the RRP value in MetaboWeiz was maximal for all 14 retrieved metabolites (that is, the true candidate was always ranked first) a mean RRP score of 0.16 for the 15 retrieved metabolites was obtained in Progenesis QI (that is, in six cases the true hit was not ranked first, causing a selection of a false hit and a decrease in the overall software recall rate). Here we report the generation of WEIZMASS, a large and structurally diverse library of high-resolution MS spectra obtained from more than 3,300 authentic standard compounds. The WEIZMASS collection mostly represents structures of plant-specialized/secondary metabolites. Complementary computational tools developed through this work will allow the construction of similar spectral libraries and their interrogation with high confidence using a consistent quantitative approach. We estimate that a single analysis of extracts derived from any given plant species using the newly developed computational and experimental methods can result in a positive identification of 30–40 metabolites from the WEIZMASS library. On the basis of botanical origin analysis of identified metabolites, all identified metabolites are shown to originate from very diverse plant genera ( Supplementary Fig. 16 ), representing the wide botanical origin of the WEIZMASS library. In addition, many of these identified metabolites will likely be either identified for the first time in the particular plant species or family investigated and in some cases never published in plants or any organism. We expect this approach to be expedient for both exotic, non-model species such as ones from the Lemnaceae family investigated here, as well as classical model plant species including A. thaliana and tomato. While current plant MS-based metabolomics reference data are mostly composed of putative or low-confidence identified metabolites, highly confident, validated metabolite identification as conducted here includes several fundamental advantages. In combination with additional biological data, highly specific identification of specialized metabolite can be an extremely powerful tool for the elucidation of metabolic pathways in any metabolism, including plants. It provides essential information with respect to likely enzyme candidates for certain reactions, including hints on substrate and product specificity and chemical substitutions positions, which would not be possible with putative assignments. It could also aid in elucidating the metabolic diversification of pathways within a genus. This study also raised a new hypothesis suggesting that some sections of the so-called ‘specialized metabolism’ might be much more common across the plant kingdom than is currently assumed. Our results point to this notion, as most of the metabolites identified here originate from very diverse and distant plant species. For example, the monoacyl-di-galactosylglycerol Gingerglycolipid A (PubChem CID45782905), which was confidently identified in both the model plant A. thaliana and members of the Lemnaceae family, was previously isolated and detected only in oriental medicinal plants such as maidenhair tree ( Ginkgo biloba ), ginger ( Zingiber officinale ) [37] and rock pine ( Orostachys japonicus ), and is utilized in traditional remedies possessing some investigated pharmaceutical applications [38] . We hope that additional, large-scale spectral libraries generated from authentic standards of plant metabolites will be available in the near future using the platform presented in this study. In addition, the range of MS spectra derived from authentic standards in the WEIZMASS library can serve as a resource for computational attempts to model and predict LC–MS features and associate them with chemical properties and classes. Improved predictive in silico capacities such as automatic RT prediction, or chemical classification by spectral patterns can eventually lead, in conjugation with experimental data, to higher levels of annotation coverage and more high-confidence assignments in metabolomics studies. The integration of MatchWeiz with other metabolite annotation strategies, for example, the recently reported methods for accurate mass-time tags and chromatographic projection [27] , [39] , can offer researchers an opportunity to expand the repertoire of confidently annotated metabolites in their favourite plant species. Features of the WEIZMASS library The spectra in the WEIZMASS spectral library were generated from the ‘MEGAbolite’ collection of 3,540 natural products purchased from AnalytiCon Discovery ( http://www.ac-discovery.com ). The 3,540 metabolites in the collection were isolated from 790 plant genera distributed worldwide and structurally resolved by the vendor using HPLC and NMR. The library contains 1,785 unique chemical formulas of which 1,386 (roughly 40% of the spectra) are not present in the Dictionary of Natural Products ( www.dnp.chemnetbase.com ) and to the best of our knowledge are not associated with an organism to date. Library acquisition, sample preparation and other experimental details are given below. WEIZMASS library preparation The ‘MEGAbolite’ collection of 3,540 natural plant collection was purchased from Analyticon Discovery ( http://www.ac-discovery.com ). The 3,540 library metabolites were injected in 177 pools of 20 metabolites each. The elution order of each pool was manually planned to avoid, as possible, isomeric metabolites included in the same pool (vendor-supplied RT windows were used to predict the elution order of metabolites). Stock solutions of chemical standards were prepared directly in the vendors 96-well plates by dilution of 0.1 mg of dry matter with 500 μl of H 2 O/HCOOH/MeOH/EtOH/DMSO at different ratios (depending on the solubility of the metabolites) using a programmable liquid-handling robot (Freedom EVO, Tecan). The samples contained mixes of 20 chemical standards with different lipophilicities, which were prepared by mixing equal amounts of standards stock solutions with a final concentration of 10 μg ml −1 per chemical standard. A volume of 5 μl of the analytical sample mix were injected to LC–MS. Analysis was performed using a UPLC-QTOF system (HDMS Synapt, Waters), with the ultra performance liquid chromatography (UPLC) column connected online to a photodiode array detector and then to the MS detector as in ref. 40 , with the following modifications: the linear gradient was from 100 to 72% phase A over 22 min, from 72 to 0% phase A over 14 min, then held at 100% phase B for further 2 min; and then returned to the initial conditions (100% phase A) in 0.5 min and conditioning at 100% phase A for 1.5 min. A divert valve (Rheodyne) excluded 1.0 and 38 min from the injection. Data acquisition was performed in the MS E mode with energy ramp [28] that records an exact mass precursor and fragment ion information from every detectable component in a sample. MS E mode rapidly alternates between two functions: the first acquiring low-energy exact mass precursor ion spectra and the second acquiring elevated-energy exact mass fragment ion spectra. The collision energy was set to 4 eV for low-energy function and to 10–30 eV ramp for the high-energy function in the positive ion mode (15–35 eV in the negative ion mode). Scan time for each function was set to 0.25 s. In addition, a mixture of 15 standard metabolites, injected after each 10 samples, was used for quality control and two additional pool samples used subsequently for retention time correction were injected in the beginning and end of each analytical sequence (see ‘Preparation of complex biological matrix pools’ (superpools) below). The MS E mode with energy ramp was used to add as much of the specific fragmentation patterns of each metabolite as possible in one continuous run. A preliminary test of the ramp mode was conducted, in which library records of tandem MS/MS data were compared with ramp mode fragmentations. The test results indicated that in the majority of cases at least two of the most abundant MS/MS fragments could also be detected in the MS E mode (62% of 49 metabolites in the NI MS mode and 70% of 62 samples in the PI MS mode). In this preliminary test a decrease in peak intensities of roughly 25–30% was also observed due to the energy ramp, indicating a reduction in the dynamic range. Preparation of complex biological matrix pools A consistent and equal (1:1) extract mixture of A. thaliana leaves and tomato ( S. lycopersicum ; cv. M82) fruit red skin (termed, ‘superpools’) was used to prepare the sample pools used for computational RT correction. Extract preparation: frozen leaves of A. thaliana from 3.5-week-old wild-type Columbia-0 plants were ground and extracted with an extraction solution (80% methanol and 0.1% formic acid) at a ratio of 1:3 (w/v). Samples were sonicated for 20 min in a bath sonicator, vortexed and centrifuged for 12 min at 14,000 g , and the supernatant was filtered through 0.22 μm polyvinylidene difluoride filters. Red skin of tomato fruit was extracted using 100% methanol (1:3 (w/v)), and otherwise prepared as Arabidopsis leaves above. Automatic generation of the WEIZMASS library The method for automatic library set-up presented in this work is a continuation of our earlier work implemented in the ‘MetaDB’ R package and workflow [41] . The raw instrument data of injected pools were first converted to NetCDF format using the MassLynx Databridge ( http://www.waters.com ). The NetCDF files containing data from the first and second MS channels were then converted into data matrices using the R ( http://www.r-project.org ) packages XCMS [42] and CAMERA [43] , with specific software parameters given in Supplementary Table 6 . The pre-processing stage generated a single peak matrix for each pooled injection, containing the m / z , RT and peak intensity profiles of both the low-energy (4 eV) and high-energy (MS E mode with energy ramp) channels. Each peak table was then processed using an R script, which uses the known theoretical values of each chemical standard to estimate which of the observed peaks best corresponds with that particular chemical standard. The process is illustrated in main text Fig. 1b : vendor-supplied RT windows are first converted to an estimated RT range, in which several possible primary ions are searched. Once a putative ion peak is detected, the R package Rdisop [20] is used to decompose the isotope pattern of the detected peak. If the theoretical chemical formula of the chemical standard, or one of possible adducts, is detected in the list of potential formulas returned by Rdisop, the putative match is validated. A validated match is then followed by adding a cluster of co-eluting peaks with correlated profiles, to the principal ion, including, when present: adduct ions, lower mass fragments and the corresponding isotope peaks. Peak profile grouping and annotation of individual peaks is principally done by the R package CAMERA. The aggregated cluster of peaks is finally defined as an R list object, forming the metabolite entry in the reference library. An example of one injection pool in the two MS ionization modes and the corresponding automatic extraction results are shown in Supplementary Figs 2–3 , and Supplementary Table 2 . An example of the used format and data organization are also shown ( Supplementary Fig. 4 ). Comparison of WEIZMASS to other libraries The ReSpect DB (http://spectra.psc.riken.jp) was downloaded as text files corresponding with 8,944 spectra. The text files were text mined to extract only spectra obtained from high-resolution MS instruments. SMILES strings ( http://www.daylight.com ) were extracted from the relevant text files to determine the amount of unique chemical structures. The number of unique chemical formulas was inferred likewise. The percent of compounds originating from chemical standards were extracted from the published results [13] . The community-based GNPS database ( https://gnps.ucsd.edu ) was interrogated using downloaded libraries in the ‘mfg’ text format. The following GNPS public spectral libraries were used: the ‘PRESTWICK PHYTOCHEM’, the ‘NIH-NATURALPRODUCTSLIBRARY’, the ‘FAULKNERLEGACY’ and the ‘GNPS LIBRARY’. The SMILES strings were extracted using text mining as before and used as an indicator for the number of unique chemical structures. Entries with missing SMILES strings were considered ambiguous (in terms of chemical structure), and were removed. Likewise, entries with unreadable SMILES strings were also removed. The overlap with the WEIZMASS library was determined using chemical fingerprints and the Tanimoto similarity index, with results equal to one interpreted as identical pairs. The Spektraris library was downloaded from the authors’ website ( http://langelabtools.wsu.edu ), and only the entries having chemical structure MOL files were considered in the comparison. The number of unique compounds, and the overlap with the WEIZMASS were performed as described above. MatchWeiz computational modules The computational modules in MatchWeiz were implemented in R and form an automated software annotation tool ( Fig. 2 ). Description of the individual software modules is given in Supplementary Note 1 and in Supplementary Figs 6–12 . MatchWeiz annotation scoring model Scores resulting from the different modules were combined into a unified metabolite annotation score, based on a linear regression model. To create the scoring model, a sufficient amount of training samples had to be generated by experimental measures. Positive training samples were initially taken from a spiking experiment of 100 chemical standards from the WEIZMASS library spiked into a biological matrix and performed in the two MS ionization modes (see ‘Spiking of chemical standards into the ‘superpool’ matrix’ below). All spiked samples were then given to MatchWeiz for annotation with the WEIZMASS reference library of 3,309 chemical standards. The annotation results were then used to evaluate both the ability of MatchWeiz to correctly retrieve metabolites from a biological matrix (see ‘Evaluation of MatchWeiz retrieval rates’ in the Results section) and to train the initial scoring model. The model training details are described below. Training of the initial annotation scoring model . The software output for 175 retrieved cases of spiked chemical standards detected by MatchWeiz were summarized into a matrix containing the calculated values of the different modules and the corresponding annotation results (which in this case, all corresponded with ‘True’ annotations). Other annotation results, derived from the biological matrix into which the chemical standards were spiked, were tagged as ‘Unknown’, and were used as references when training the model. Using this training matrix, a logistic regression model was trained using the ‘glm’ function in R, with the distribution family parameter set to ‘binomial’ (‘logit’ model). The model prediction results, including both the ‘True’ and ‘Unknown’ annotations, were then analysed in an unsupervised manner by Principal Component Analysis and a dot plot ( Supplementary Fig. 13 ). According to the dot plot, >90% of the ‘True’ annotations and < 10% of the ‘Unknown’ annotations are in the predicted sum score range >0.1; therefore, the initial scoring threshold for considering a putative annotation as a true hit was set to 0.1. This initial model was then used in a series of plant species focused annotations, validated by spiking experiments and which also added more examples for retraining the scoring model. Retraining the scoring model . Metabolites that were confidently identified through the plant species experiments were used to train a new version of the annotation scoring model. The training data contained all the confirmed identifications, as well as all the false identifications, resulting in a training matrix of 620 positive examples and 482 negative examples. The training errors were calculated by 1,000-fold cross-validation: the model was iteratively trained based on a random subset of two-thirds of the data, and then tested on the remaining third. Error measures were recorded for each model and summarized after 1,000 iterations. Finally, the model was trained using the full data matrix, consisting of 1,102 examples. We next tested if adding a pair interaction of predictive variables can improve the model in terms of error rates. All possible pair interactions between the predictive variables, consisting of 28 possible pairs, were tested using the cross-validation process described above. The models with their pair interactions and the corresponding error measures are shown in Supplementary Table 7 . The preferred model, chosen by the maximum ‘F1measure’ and ‘recall’ values, includes the ‘mainIon-fragments’ interaction pair (with an ‘F1-measure’ of 0.73 and a recall of 0.72, compared with 0.71 and 0.715, respectively, for the model without any interaction). Although the improvement in test results when adding an interaction pair is small, the chosen interaction pair makes an analytical sense: the pair relates to the mutual importance of accurately matching the molecular ion together with the matching of fragment ions by the X-Rank algorithm. The final scoring model is given below. where modules are the individual outputs of the previously described software modules (that is: ‘coverage’, ‘main ion’, ‘principal ion’, ‘adducts’, ‘isotope decomposition’, ‘fragment matching’, ‘cross reference’ and ‘RT penalty’), and ‘mainIon:fragments’ the selected interaction pair. Model coefficients and summary statistics are presented in Supplementary Table 8 . Spiking of chemical standards into the superpool matrix One hundred metabolite standards were randomly selected out of the 3,309 reference library metabolites available in both MS ionization modes. The metabolites were arranged in 15 groups of six or seven chemical standards each and then spiked into the ‘superpool’ matrix described before. The final concentration of the chemical standards was about 7 μg ml −1 each. Experimental LC–MS analysis, data conversion and computational preprocessing were done as described above `WEIZMASS library preparation', using the same parameters. Identification of metabolites in three plant species MatchWeiz, coupled to the WEIZMASS library was used to annotate peaks obtained by analysing extract derived from three plant species: A. thaliana (ecotype Col.), members of the Lemnaceae family and tomato ( S. lycopersicum; cv. Micro Tom). The preprocessing of the raw data for the three plant species was done as described above (the ‘WEIZMASS library preparation’), with the only exception that raw samples were preprocessed in groups according to the relevant experimental groups (that is, biological tissues and conditions). Experimental details and LC–MS injection data of plant tissues for annotation and validation are given below. Sample preparation of plant tissues for validation A. thaliana plants (ecotype Col-0 ) were grown as described in Bocobza et al . [44] . Nine plant tissues were analysed including young and mature leaves (12 days, 3–4 weeks and 6–7 weeks after sowing, respectively), inflorescence and inflorescence leaves, closed buds, open flowers and siliques in two development stages (1 and 2 cm lengths). Sample preparation was done as described in `Preparation of complex biological matrix pools' (superpools) for A. thaliana , above. Tomato plants ( S. lycopersicum cv. Microtom) were grown as described in Itkin et al . [45] . The following tomato tissues were analysed: fruit skin and flesh in five developmental stages (immature green, mature green, breaker, orange and red fruit), leaves (young and mature), buds, flower buds, open flowers, pollen and roots. Sample preparation was done as described in `Preparation of complex biological matrix pools' (superpools) for tomato, above. Plants of several genus of the Lemnaceae family ( L. gibba , S. polyrhiza and S. oligo ( L. punctata )) were grown as described earlier [46] . In the case of L. gibba tissues, the plants were transferred to Petri dishes followed by manual separation of mature, young and rhizome plant parts. Sample preparation was done as described in ‘Preparation of complex biological matrix pools’ (superpools) for A. thaliana , above. For annotation validations by spiking into plant tissues, three samples were prepared for consecutive injections: the plant tissue containing the endogenous metabolites; the spikes of the relevant chemical standard into the corresponding plant matrix; and a mix of four or five of the relevant pure chemical standards. The plant tissues were diluted, respectively, with an extraction buffer to compensate for the change in concentration resulting from the addition of the chemical standards. Spiked samples were prepared by mixing of plant extract (80 μl) with the mix of standards (20 μl). The pure plant tissue was prepared by mixing of plant extract (80 μl) with dilution solution (20 μl). The pure mix of chemical standards was prepared by mixing of dilution solution (80 μl) with the mix of standards (20 μl). Determining the novelty of identified metabolites We examined each identified metabolite found in the three investigated plant species (31 in Lemnaceae, 40 in tomato and 38 in Arabidopsis ) to set its degree of novelty. The metabolites comprising the WEIZMASS library are not novel in terms of structure identification but possess novelty in terms of association to a specific organism, to plants, plant family, genus or species. We defined ‘not novel’ as metabolites that were detected and published before for the specific plant species; ‘never reported in the plant species’ as metabolites that were detected and published in other plants, but not in the particular plant species or genus; and ‘never published’ for metabolites where no publication was found that describes the detection of that metabolite in any organism. The metabolites identified in tomato were first screened against an in-house list of known LC–MS-detected tomato metabolites. Next, the metabolites that did not match any item in the in-house list were searched against public reference databases using the SciFinder system ( http://www.cas.org ). The search was done either by using the metabolite name or by using the chemical structure. Stereo-chemistry, when available, was kept, otherwise, all available tautomers were considered. All results of the literature search, when available, were next filtered by the species name and the resulting references were checked manually to examine if the query metabolite was identified in the plant species. A single reference was retained from the search results, if found, and added to the summary tables ( Supplementary Data 1–3 ). In cases where after filtering no references were found, the metabolite was considered as ‘never reported in that plant species’, while metabolites with no references at all were considered as ‘never published or associated with any organism’, obviously any plant species. Likewise, for A. thaliana , the identified library metabolites were first searched against an in-house reference list and the AraCyc public database ( http://www.plantcyc.org ) and the remaining metabolites were checked using the SciFinder system as for tomato above. The identified library metabolites in members of the Lemnaceae family were checked using the SciFinder system only. Clustering of identified metabolites by structural similarity SMILES strings ( http://www.daylight.com ) of the identified library metabolites were converted from the SDF data obtained from the vendor using the Open Babel chemical toolbox [47] . The R package ‘Rcdk’ [48] was used to calculate pairs of Tanimoto similarity index between molecular structures and to generate the derived similarity matrix [26] . The similarity matrix was then used to make a structural ‘chemical-tree’ based on hierarchical clustering by similarity values. The R package ‘ape’ with the tree type set to ‘unrooted’ was finally used for plotting the clusters. Clustering of chromatographic peaks by intensity profiles A peak list matrix containing the entire experimental LC–MS data for each plant was first generated using the ‘xcms’ and ‘CAMERA’ R packages, as described above. The integrated peak areas were then averaged column-wise between technical repeats of the same biological tissue, leaving a matrix with a reduced column size. The natural log values were then taken and the resulting log-transformed matrix was summed up row-wise according to the peak clusters (pcgroups) detected by the CAMERA package. This resulted in a matrix with a reduced the row size, where each row is the summed up log values (‘logI’) of several co-eluting peaks, which belong to the same cluster group. Apart from simplifying the presentation, the above procedure reduces the complexity of the data by relating several LC–MS features to one or several chemical entities (that is, metabolites, many of them unknown). We next mapped the identified library metabolites into the matrix by their CAMERA ‘pcgroups’ indices and then performed hierarchical clustering by intensity profiles on the whole matrix. In the case of A. thaliana , an extra set of putatively identified metabolites, detected in earlier studies, were also mapped into the matrix ( Fig. 6 ), in order to put the newly identified metabolites in the context of known ones. The data was finally plotted using the ‘heatmap.2’ function in R, and clusters of interest containing both the identified library metabolites and known ones were selected and described in detail ( Fig. 6b,c ). Analysis of identified metabolites by botanical origin The taxonomy lineage of 671 plant genera, corresponding with the botanical origin of the majority of metabolites in the WEIZMASS library, was downloaded from the NCBI taxonomy browser ( http://www.ncbi.nlm.nih.gov/taxonomy ) in the PHYLIP (Newick) format. Next, the taxonomy tree was read and printed as an outline by the R package ‘ape’, with the tree type set to ‘unrooted’. Tree tip labels corresponding with the plant genera of identified metabolites were overlaid on top of the unrooted tree. The number of matching plant genera in each of the plant species were as follows: 26 (out of 31 identifications) in Lemnaceae; 39 (out of 40 identifications) in tomato; and 35 (out of 38 identifications) in A. thaliana . The botanical origin by plant genera of metabolites in the WEIZMASS library was supplied by the vendor (Analyticon Discovery Company). Chemical structures of identified metabolites can be found in Supplementary Data 7 . Comparison of MatchWeiz to other software The ‘naive’ algorithm was implemented as a simple search by RT and mass-to-mass matching using tunable tolerance values. The initial settings, set by the instrument’s specifications, were ±2% allowed deviation in RT and a 5 p.p.m. deviation in m / z , relative to the values registered in the library. Next, more liberal settings of ±60 s allowed deviation in RT and 15 p.p.m. deviation in m / z were used. A minimum group of two or three matching peaks for an annotation were required for the NI and PI modes, respectively. Data for comparison were acquired on a UPLC-QTOF model (a XEVO G2-S, Waters), to match the designated specifications of Progenesis QI (http://www.nonlinear.com ). Tomato fruit skin samples (two biological replicates) were used, as described above (‘Sample preparation of plant tissues for validation’). The instrumental set-up of the UPLC-QTOF was as described in the WEIZMASS library preparation section, apart from the shorter chromatographic gradient (26 min). All software (that is MatchWeiz, the ‘naive’ search and Progenesis QI) were given the same input data and the resulting retrieval rates were calculated based on available experimentally validated results (that is: confirmed identifications in tomato skin tissues), composed of 15 metabolites that were identified in this study. The outputs of MatchWeiz and Progenesis QI were filtered using a threshold set to 50% of the maximum respective annotation score, and in cases of multiple annotations corresponding with the same group of peaks, only the highest scoring candidate was taken. For MatchWeiz, this approach implied a 0.5 score threshold, while in Progenesis QI a score of 40 was used based on a maximum score of 80 (as ion-mobility data were not available, 20 points were deducted from the maximum score of 100). Next, the RRP [36] was calculated for each identified metabolite, using the sorted list of candidate scores coming from each software after filtering by the threshold score. The sums of candidates coming from each software was likewise calculated after removing candidates below the set score threshold and taking the remaining candidates corresponding with each peak group (MatchWeiz and Progenesis QI). For the ‘naive’ search method, the unsorted sums of candidates were considered, and no RRP was calculated, as annotation scores were not calculated. Data availability statement The MatchWeiz software and computational methods required to create the WEIZMASS library have been implemented as an R package available on GitHub ( https://github.com/AharoniLab/MatchWeiz ). Raw LC–MS data of plant material supporting metabolite findings in this study were deposited in the MetaboLights repository ( http://www.ebi.ac.uk/metabolights/MTBLS330 ). The authors declare that all other data supporting the findings of this study including the WEIZMASS library spectra can be made available for academic use on request from the corresponding author. How to cite this article: Shahaf, N. et al . The WEIZMASS spectral library for high-confidence metabolite identification. Nat. Commun. 7:12423 doi: 10.1038/ncomms12423 (2016).